IκBβ enhances the generation of the low-affinity NFκB/RelA homodimer The NFκB family of dimeric transcription factors regulate inflammatory and immune responses. While the dynamic control of NFκB dimer activity via the IκB–NFκB signalling module is well understood, there is little information on how specific dimer repertoires are generated from Rel family polypeptides. Here we report the iterative construction—guided by in vitro and in vivo experimentation—of a mathematical model of the Rel-NFκB generation module. Our study reveals that IκBβ has essential functions within the Rel-NFκB generation module, specifically for the RelA:RelA homodimer, which controls a subset of NFκB target genes. Our findings revise the current dogma of the three classical, functionally related IκB proteins by distinguishing between a positive ‘licensing’ factor (IκBβ) that contributes to determining the available NFκB dimer repertoire in a cell’s steady state, and negative feedback regulators (IκBα and -ɛ) that determine the duration and dynamics of the cellular response to an inflammatory stimulus. The NFκB family of dimeric transcription factors are known to control the development, maturation and responses of the immune system comprising diverse cell types. Resting, unstimulated cells contain a latent pool of NFκB dimers in the cytosol that are stoichiometrically associated with their inhibitors, the IκBs [1] , [2] . NFκB transcription factors are produced by homo- or heterodimerization from a pool of five Rel homology domain-containing proteins (RelA, RelB, cRel, p50 and p52). The IκB family comprises several isoforms including the classical IκBα, IκBβ, IκBɛ proteins and the IκBγ and IκBδ activities contained within the higher molecular weight IκBsome [3] . Combinatorial dimerization and IκB–NFκB interactions are hallmarks of the IκB–NFκB signalling system. The coordinated functions of IκB proteins in controlling the dynamics of NFκB activity have been studied systematically using a combined experimental and mathematical modelling approach. Specifically, mathematical modelling recapitulates the key mechanisms, such as stimulus-responsive, IκB kinase (IKK)-dependent degradation of IκBs, release of nuclear NFκB DNA-binding activity, as well as subsequent attenuation via the negative feedback regulators IκBα, IκBɛ, A20 and IκBδ (ref. 4 ). Interestingly, these studies did not identify a critical function for IκBβ, and IκBβ-deficient mice and cells show attenuated, not increased inflammatory responses [5] . In contrast, little recent progress has been reported on how NFκB dimers are generated. Early studies led to an appreciation that the NFκB transcription factor family consists of up to 15 possible dimers, and that different dimers are detectable in different cell types [1] . In fact, the NFκB dimer repertoire changes dramatically during cell differentiation; for example, B-cell lines with early lineage markers contain primarily RelA:p50, while those with later lineage markers contain primarily cRel:p50 dimers [6] . In murine embryonic fibroblasts (MEFs), the RelA:p50 heterodimer and the RelA:RelA homodimer have been observed and shown to be responsible for the expression of distinct target genes [7] . Indeed, despite its much lower abundance in fibroblasts, the RelA:RelA homodimer was shown to have nonredundant functions for a subset of NFκB target genes, with the specificity being mediated by κB-site DNA sequences as well as transcriptional co-activators [8] . However, surprisingly little is known about the mechanisms that control the formation of these distinct NFκB dimers that are critical for mediating gene-specific expression control. Indeed, we presently lack a quantitative understanding of the most fundamental processes of monomer synthesis and subsequent dimer formation. Here we have employed mathematical modelling and experimental approaches iteratively to study the mechanisms that control the fibroblast-specific NFκB dimer repertoire. Guided by a model based on first principles of protein–protein interactions, and using in vitro biophysical interaction measurement, we found that we can only account for the in vivo observations of low-affinity dimers when we considered additional mechanisms. Specifically, combined experimental and computational studies revealed that IκBβ functions as a positive regulator within the Rel-NFκB dimer generation module, and is essential for the formation of RelA:RelA homodimers. In contrast, IκBα is the key regulator of the dynamics of NFκB activity, not only of RelA:p50 but also of RelA:RelA. We conclude that the classical IκBs actually fall into two classes; whereas IκBα and -ɛ primarily function within the IκB–NFκB signalling module that is responsive to inflammatory stimuli, IκBβ primarily functions within the Rel-NFκB dimer generation module. The resulting model not only recapitulates experimental observations, but also explains the contrasting phenotypes of mice deficient for each of the classical IκBs. NFκB dimerization affinities and monomer competition To address the molecular basis for the generation of a MEF-specific repertoire of NFκB dimers within the so-called ‘Rel-NFκB dimer generation module’, we first considered the fundamental principles pertaining to the generation of homo- and heterodimers from the classical NFκB proteins p50 (50) and RelA (A), which are present in all differentiated human cells, and which show distinct gene-expression specificities [7] , [8] . Dimer abundance may be thought of as a function of monomer synthesis ( m 1 , m 2 ) and degradation ( m −1 , m −2 ), and combinatorial dimer association ( d 1 , d 2 , d 3 ) and dissociation (d −1 , d −2 , d −3 ) rate constants ( Fig. 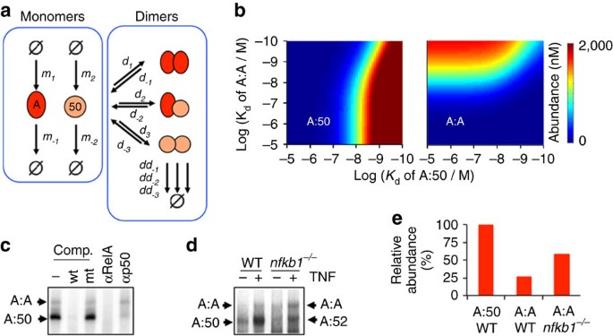Figure 1: Monomer competition reduces the abundance of the RelA homodimer. (a) A schematic of a simple model depicting the dimerization of NFκB RelA and p50 polypeptides.m1andm2are synthesis rate constants,m−1andm−2are degradation rate constants.d1, d2andd3are dimer association rate constants, whiled−1, d−2andd−3are dimer dissociation rate constants.dd−1,dd−2anddd−3are dimer degradation rate constants. (b) Heat maps of protein abundances of A:A and A:50 dimers computationally simulated as a function of the dimer affinities (Kd). These were generated by the model schematized ina. (c) Electrophoretic mobility shift assays (EMSA) with nuclear extracts prepared from TNF-stimulated (30 min) wild-type MEFs. The identity of the indicated DNA–protein complexes were confirmed using competition (comp.) with a 100-fold excess of unlabelled double-stranded oligonucleotide that either contains the wild-type (wt) or mutant (mt) κB site sequence. The RelA and p50 antibodies (α–RelA and α-p50) are used in shift-ablation studies to confirm that the identity of the A:A-DNA and A:50-DNA complexes. (d) EMSA with nuclear extracts prepared from TNF-stimulated (30 min) wild-type andnfkb1−/−MEFs. (e) Bar graph comparison of the abundances of A:A NFκB dimers wild-type andnfkb1−/−relative to the wild-type A:50 bands (100%) fromd. 1a , Supplementary Table 1 , Supplementary Note 1 ). As RNAseq data show very similar absolute abundances of the RelA and p50-encoding mRNAs in wild-type MEFs ( Supplementary Fig. 1a ), the synthesis rates of the protein monomers are assumed to be equal in the model. As Rel proteins are obligate dimers, monomers are incompletely folded and more rapidly degraded in vivo than when dimerized ( dd −1 , dd −2 , dd −3 ) [9] , [10] . Figure 1: Monomer competition reduces the abundance of the RelA homodimer. ( a ) A schematic of a simple model depicting the dimerization of NFκB RelA and p50 polypeptides. m 1 and m 2 are synthesis rate constants, m −1 and m −2 are degradation rate constants. d 1 , d 2 and d 3 are dimer association rate constants, while d −1 , d −2 and d −3 are dimer dissociation rate constants. dd −1 , dd −2 and dd −3 are dimer degradation rate constants. ( b ) Heat maps of protein abundances of A:A and A:50 dimers computationally simulated as a function of the dimer affinities (Kd). These were generated by the model schematized in a . ( c ) Electrophoretic mobility shift assays (EMSA) with nuclear extracts prepared from TNF-stimulated (30 min) wild-type MEFs. The identity of the indicated DNA–protein complexes were confirmed using competition (comp.) with a 100-fold excess of unlabelled double-stranded oligonucleotide that either contains the wild-type (wt) or mutant (mt) κB site sequence. The RelA and p50 antibodies (α–RelA and α-p50) are used in shift-ablation studies to confirm that the identity of the A:A-DNA and A:50-DNA complexes. ( d ) EMSA with nuclear extracts prepared from TNF-stimulated (30 min) wild-type and nfkb1 −/− MEFs. ( e ) Bar graph comparison of the abundances of A:A NFκB dimers wild-type and nfkb1 −/− relative to the wild-type A:50 bands (100%) from d . Full size image Dimerization affinities are the key determinants of cellular homo- and heterodimer abundances. We simulated the abundance of RelA:RelA (A:A) and RelA:p50 (A:50) dimers as a function of those dimer affinities keeping the p50:p50 dimer affinity constant at 30 nM ( Fig. 1b ), 3 and 300 nM ( Supplementary Fig. 1b ). Whereas p50:p50 dimerization affinity did not affect A:A or A:50 abundances over that range, the simulations do illustrate an interdependence between A:A and A:50 formation, whereby p50 competes for RelA monomers and may thus inhibit A:A generation. To test whether monomer competition occurs in cells, we compared nfkb1 −/− (which lack p50) and wild-type MEFs and found an increase in the abundance of the A:A homodimers. These data support the concept that monomer competition is physiologically relevant and tends to diminish the abundances of weaker affinity dimers ( Fig. 1c–e ). To parameterize the model, we next measured dimer affinities with biophysical techniques. Homodimer affinities were measured by analytical ultracentrifugation using purified recombinant RelA and p50 dimerization domains ( Supplementary Fig. 1c ). The heterodimer affinity was deduced from quantitative gel filtration experiments that provided the ratios of dimer abundances ( Supplementary Fig. 1d–f ). We found remarkably disparate affinities: whereas the interactions by p50 proteins were found within the expected range (5–40 nM), the A:A homodimer affinity was in the μM range ( Fig. 2a ). Employing these rate constants in the kinetic model resulted in the prediction that the A:A homodimers would have exceedingly low abundance (<4% of total RelA-containing dimers) because of a weak A:A affinity and the above-described monomer competition. However, testing this prediction experimentally, we found that A:A homodimers were readily detectable in cells amounting to about a quarter of tumour-necrosis factor (TNF)-inducible NFκB activities ( Fig. 2b ). Thus, the mismatch between model prediction and experimental results suggested that there might be additional mechanisms controlling dimer abundance that are not included in this version of the kinetic model. 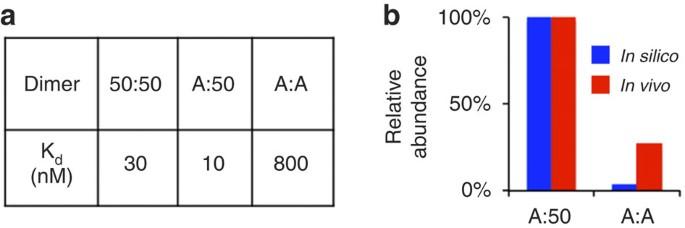Figure 2: Biophysical kinetic model underestimates the abundance of the RelA homodimer. (a) Summary table of dimer affinities as measured with AUC and quantitative gel-filtration analysis of purified recombinant proteins (Supplementary Fig. 1b–e). The A:A homodimer affinity is lower than those of p50-containing dimers. (b) The bar graph is a quantitation fromFig. 1showing a comparison of model predicted (blue) and experimentally measured (red) relative abundances of A:A and A:50 dimers. Figure 2: Biophysical kinetic model underestimates the abundance of the RelA homodimer. ( a ) Summary table of dimer affinities as measured with AUC and quantitative gel-filtration analysis of purified recombinant proteins ( Supplementary Fig. 1b–e ). The A:A homodimer affinity is lower than those of p50-containing dimers. ( b ) The bar graph is a quantitation from Fig. 1 showing a comparison of model predicted (blue) and experimentally measured (red) relative abundances of A:A and A:50 dimers. Full size image Interaction affinities between IκB isoforms and NFκB dimers Given that IκBs associate along a large dimerization interface [11] , and NFκBs interacting with IκBs protect the latter from degradation [12] , [13] , [14] , we considered the possibility that IκBs may stabilize RelA-containing NFκB dimers. (Classical IκBs do not interact with p50:p50 (ref. 15 ).) To test this idea, we extended the mathematical model by including IκB synthesis ( i 1 ) and degradation ( i -1 ) and its interaction with A:A homodimers and A:50 heterodimers ( di 1 , di −1 , di 2 , di −2 ; Fig. 3a , Supplementary Table 2 , Supplementary Note 2 ). In the resulting model, NFκB dimer abundances are then also a function of IκB abundances and the interaction affinities between NFκB dimers and IκB proteins. These interactions are thought to be tight; [12] , [16] , [17] however, systematic measurements using biophysical methods are hampered by the challenge of expressing and purifying full-length recombinant proteins that are not fully folded in the apo-form and have a tendency to aggregate. 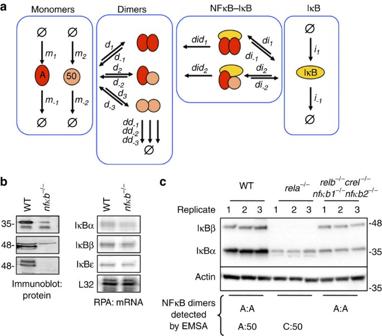Figure 3: Differential interaction affinities for IκB and NFκB family members. (a) A model schematic of the Rel-NFκB dimer generation module. It depicts the dimerization of RelA and p50 NFκB polypeptides as inFig. 1a, with the addition of a prototypical inhibitor of NFκB (IκB).m1andm2are RelA and p50 synthesis rate constants,m−1andm−2are RelA and p50 degradation rate constants, respectively.d1, d2andd3are dimer association rate constants, whiled−1, d−2andd−3are A:A, A:p50 and p50:p50 dimer dissociation rate constants, respectively.dd−1,dd−2anddd−3are A:A, A:p50 and p50:p50 dimer degradation rate constants, respectively.i1is the IκB synthesis rate constant,i−1is the IκB degradation rate constant.di1and di2are the IκB–NFκB association rate constants.Di−1anddi−2are the IκB–NFκB dissociation rate constants.did1anddid2are the IκB–NFκB degradation rate constants of IκB to release NFκB. (b) Immunoblot (left panel) of whole-cell extracts of wild-type MEFs and MEFs deficient in canonical NFκB genes (RelA, cRel and p50) using antibodies against the indicated proteins (IκBα, IκBβ and IκBɛ). RNAse protection assay (RPA, right panel) of previous extracts to measure transcript levels of the indicated genes (IκBα, IκBβ, IκBɛ and L32). Immunoblot and RPA data are representative of more than three independent experiments that consistently show a deep reduction IκB protein levels without a corresponding reduction in transcript levels. (c) Immunoblot of indicated IκBs in indicated NFκB dimer compound knockout MEFs as compared to wild type MEFs, with the indicated NFκB dimers below. The blot is a representative of three independent experiments that consistently showed that presence of RelA is required and sufficient for the detection of IκBβ protein. Quantitation of this data is shown as bar graphs inFig. 4a. Figure 3: Differential interaction affinities for IκB and NFκB family members. ( a ) A model schematic of the Rel-NFκB dimer generation module. It depicts the dimerization of RelA and p50 NFκB polypeptides as in Fig. 1a , with the addition of a prototypical inhibitor of NFκB (IκB). m 1 and m 2 are RelA and p50 synthesis rate constants, m −1 and m −2 are RelA and p50 degradation rate constants, respectively. d 1 , d 2 and d 3 are dimer association rate constants, while d −1 , d −2 and d −3 are A:A, A:p50 and p50:p50 dimer dissociation rate constants, respectively. dd −1 , dd −2 and dd −3 are A:A, A:p50 and p50:p50 dimer degradation rate constants, respectively. i 1 is the IκB synthesis rate constant, i −1 is the IκB degradation rate constant. di 1 and di 2 are the IκB–NFκB association rate constants. Di −1 and di −2 are the IκB–NFκB dissociation rate constants. did 1 and did 2 are the IκB–NFκB degradation rate constants of IκB to release NFκB. ( b ) Immunoblot (left panel) of whole-cell extracts of wild-type MEFs and MEFs deficient in canonical NFκB genes (RelA, cRel and p50) using antibodies against the indicated proteins (IκBα, IκBβ and IκBɛ). RNAse protection assay (RPA, right panel) of previous extracts to measure transcript levels of the indicated genes (IκBα, IκBβ, IκBɛ and L32). Immunoblot and RPA data are representative of more than three independent experiments that consistently show a deep reduction IκB protein levels without a corresponding reduction in transcript levels. ( c ) Immunoblot of indicated IκBs in indicated NFκB dimer compound knockout MEFs as compared to wild type MEFs, with the indicated NFκB dimers below. The blot is a representative of three independent experiments that consistently showed that presence of RelA is required and sufficient for the detection of IκBβ protein. Quantitation of this data is shown as bar graphs in Fig. 4a . Full size image To address this challenge, we developed an approach to derive in vivo IκB–NFκB affinities. The fact that IκBα, IκBβ and IκBɛ protein abundances in MEFs deficient in classical NFκB dimers ( rela −/− crel −/− nfkb1 −/− ) were much more reduced than their corresponding mRNA levels ( Fig. 3b ) indicated the degree to which the interaction with NFκB stabilized the half-life of the three classical IκBs as established by previous reports [12] , [14] . We reasoned that measurements of relative abundances of IκB proteins in mutant cells with alternate NFκB dimer repertoires could be used to infer in vivo IκB–NFκB dimer affinities. To distinguish IκB interaction affinities for the A:50 and A:A dimers, we produced composite NFκB knockout MEFs ( relb −/− nfkb2 −/− nfkb1 −/− crel −/− ) in which RelA is the sole NFκB protein family member, and RelA-deficient MEFs, which do not contain A:A homodimers but contain the partially compensating cRel:p50 heterodimer in place of A:50 (refs 7 , 18 ; Supplementary Fig. 2a,b ). Using these cells, the experimentally determined IκBα/IκBβ abundance ratios ( Fig. 3c ) constrained the acceptable ranges of IκB–NFκB affinities via model parameter fitting procedures ( Fig. 4a ). For example, in A:50-deficient cells, the IκBα abundance was reduced to 35±8% of that in wild-type cells, constraining the IκBα-A:A and IκBα-A:50 affinity to a narrow band within the two-dimensional parameter space (top left panel). In contrast, IκBβ abundance was hardly affected (76±24% of the wild-type cells) and provided less constraint on the acceptable affinities of IκBβ-A:A and IκBβ-A:50 interactions on the basis of the particular parameter landscape (top right panel). Similarly, IκBα and IκBβ abundance measurements in A:A-deficient cells provided additional constraints (bottom panels). The overlap of these acceptable ranges for each IκB in both NFκB knockout conditions determined not a single parameter set, but rather a narrower range of parameters that can account for all available experimental data. 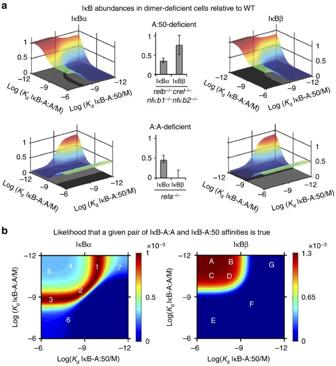Figure 4: Deriving probable IκB–NFκB interaction affinities from experimental data. (a) Surface plots of indicated IκB abundances (-α or -β) in cells deficient for the indicated NFκB dimer (RelA:p50 heterodimer-deficient, top; RelA:RelA homodimer-deficient, bottom) over the indicated ranges of IκB–NFκB affinities, as predicted by the model schematized inFig. 3a. Middle, bar graphs of the experimentally IκB abundances in the indicated NFκB dimer-deficient cells relative to WT. (A representative data figure is shown inFig. 3c.) Experimentally determined abundances constrained the range of allowable IκB–NFκB affinities in the surface plots, indicated by shadows on thexyplane. (b) Heat maps of probable IκB–NFκB affinities. Probabilities (indicated in the colour scale) were calculated using the distribution experimental measurements, defined by the mean and s.d. (Figs 2a,3cand4a); they describe the relative likelihood that an indicate parameter set if correct based on available experimental data. The most probable IκB–NFκB affinities are in red, while the least probable affinities are in dark blue. Selected probable and improbable parameter values are indicated (white letters and numbers, listed inSupplementary Table 5), and were used for model predictions inFig. 5. Figure 4: Deriving probable IκB–NFκB interaction affinities from experimental data. ( a ) Surface plots of indicated IκB abundances (-α or -β) in cells deficient for the indicated NFκB dimer (RelA:p50 heterodimer-deficient, top; RelA:RelA homodimer-deficient, bottom) over the indicated ranges of IκB–NFκB affinities, as predicted by the model schematized in Fig. 3a . Middle, bar graphs of the experimentally IκB abundances in the indicated NFκB dimer-deficient cells relative to WT. (A representative data figure is shown in Fig. 3c .) Experimentally determined abundances constrained the range of allowable IκB–NFκB affinities in the surface plots, indicated by shadows on the xy plane. ( b ) Heat maps of probable IκB–NFκB affinities. Probabilities (indicated in the colour scale) were calculated using the distribution experimental measurements, defined by the mean and s.d. ( Figs 2a , 3c and 4a ); they describe the relative likelihood that an indicate parameter set if correct based on available experimental data. The most probable IκB–NFκB affinities are in red, while the least probable affinities are in dark blue. 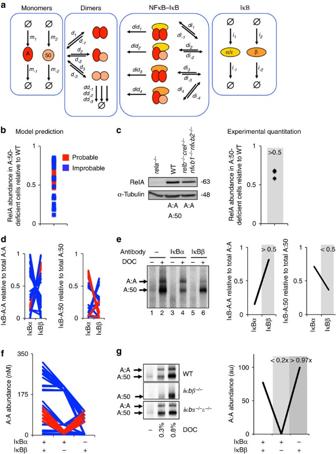Figure 5: Iterative testing and refinement of the IκBβ-RelA homodimer preference model. (a) A model schematic of the Rel-NFκB dimer generation module, as inFig. 3abut with two IκBs, IκBα and IκBβ, necessitatingi1andi2synthesis rate constants,i−1andi−2degradation rate constants,di1,di2,di3anddi4IκB–NFκB association rate constants.di−1,di−2, di−3anddi−4IκB–NFκB dissociation rate constants, anddid1, did2, did3anddid4IκB–NFκB degradation rate constants of IκB to release NFκB. (b) Computational prediction of RelA protein abundance in A:50-deficient cells (relative to wild-type cells), using probable (red) and improbable (blue) affinities shown inFig. 4band listed inSupplementary Table 5. (c) Immunoblot against RelA of whole-cell extracts from RelA-deficient, wild type and RelA-only MEFs. The right panel shows the quantitation of three independent experiments. These consistently showed values of >0.5. (d) Computational predictions of the abundances of NFκB dimers RelA:RelA (left) and RelA:p50 (right) bound to either IκBα or IκBβ as indicated. These calculations used probable (red) and improbable affinities (blue) as inb. (e) EMSA of DOC-treated cytoplasmic extracts (which results in the separation of NFκB dimers from IκBs) to quantitate IκB-bound NFκB dimer abundance. Prior immunodepletion of the extracts with antibodies against IκBα or IκBβ allows quantitation of NFκB bound to the remaining IκB isoform. Data shown are representative of three independent experiments, and the right panel shows the corresponding quantitation. (f) Computational predictions of the basal abundances of the RelA:RelA homodimer in wild-type, IκBβ-deficient and IκBα-deficient MEFs using probable (red) and improbable (blue) affinities as inb. (g) EMSAs (left panel) of DOC-treated cytoplasmic extracts of wild-type, IκBβ-deficient and IκBα/ɛ-deficient MEFs. Shown is a representative result of three independent experiments, and the right panel shows the corresponding quantitation. Selected probable and improbable parameter values are indicated (white letters and numbers, listed in Supplementary Table 5 ), and were used for model predictions in Fig. 5 . Full size image As the NFκB dimer affinity and IκB abundance measurements are associated with experimental error, we sought to characterize the resulting uncertainty about the true IκB–NFκB affinities. To do so, we calculated a probability for each IκB abundance on the basis of a twofold variance around the mean of NFκB affinity measurements. Then, we compared these values to the experimentally determined distributions (defined by mean and s.d.) of IκB abundances. This allowed us to determine the likelihood that a given pair of IκB-A:A and IκB-A:50 affinities is true based on all available experimental data along with its associated uncertainty ( Fig. 4b ). This analysis allowed us to define the ranges of probable IκB-dimer affinities and it demonstrated that IκBβ was consistently predicted to have a clear preference for A:A over A:50 (>100-fold). We chose seven parameter sets as representatives of the probable and improbable parameter spaces governing IκBα and IκBβ interactions ( Fig. 4b , Supplementary Table 5 ) in order to ascertain their likelihood in further cell biological assays. Testing the model of IκBβ controlling the RelA homodimer Using the combination of probable and improbable parameter sets ( Supplementary Table 5 ) for IκB–NFκB dimer affinities within the experimentally determined ranges, we parameterized a mathematical model to account for the generation of distinct RelA dimers ( Fig. 5a , Supplementary Table 3 , Supplementary Note 3 ). We developed three predictions that depend on high IκBβ preference for the A:A homodimer and tested them experimentally. First, we used the model to calculate the basal abundance of RelA protein in cells containing only RelA ( relb −/− nfkb2 −/− nfkb1 −/− crel −/− ) under two regimes, probable and improbable affinity predictions ( Supplementary Table 5 ). We found that most probable affinity sets predicted a lower decrease ( ∼ 1.5- to 2-fold) in RelA protein levels than most improbable affinity sets ( Fig. 5b ). Indeed, immunoblot analysis showed only a small decrease ( ∼ 1.5-fold) in RelA protein ( Fig. 5c ). Figure 5: Iterative testing and refinement of the IκBβ-RelA homodimer preference model. ( a ) A model schematic of the Rel-NFκB dimer generation module, as in Fig. 3a but with two IκBs, IκBα and IκBβ, necessitating i 1 and i 2 synthesis rate constants, i −1 and i −2 degradation rate constants, di 1 ,di 2 , di 3 and di 4 IκB–NFκB association rate constants. di −1 , di −2 , di −3 and di −4 IκB–NFκB dissociation rate constants, and did 1 , did 2 , did 3 and did 4 IκB–NFκB degradation rate constants of IκB to release NFκB. ( b ) Computational prediction of RelA protein abundance in A:50-deficient cells (relative to wild-type cells), using probable (red) and improbable (blue) affinities shown in Fig. 4b and listed in Supplementary Table 5 . ( c ) Immunoblot against RelA of whole-cell extracts from RelA-deficient, wild type and RelA-only MEFs. The right panel shows the quantitation of three independent experiments. These consistently showed values of >0.5. ( d ) Computational predictions of the abundances of NFκB dimers RelA:RelA (left) and RelA:p50 (right) bound to either IκBα or IκBβ as indicated. These calculations used probable (red) and improbable affinities (blue) as in b . ( e ) EMSA of DOC-treated cytoplasmic extracts (which results in the separation of NFκB dimers from IκBs) to quantitate IκB-bound NFκB dimer abundance. Prior immunodepletion of the extracts with antibodies against IκBα or IκBβ allows quantitation of NFκB bound to the remaining IκB isoform. Data shown are representative of three independent experiments, and the right panel shows the corresponding quantitation. ( f ) Computational predictions of the basal abundances of the RelA:RelA homodimer in wild-type, IκBβ-deficient and IκBα-deficient MEFs using probable (red) and improbable (blue) affinities as in b . ( g ) EMSAs (left panel) of DOC-treated cytoplasmic extracts of wild-type, IκBβ-deficient and IκBα/ɛ-deficient MEFs. Shown is a representative result of three independent experiments, and the right panel shows the corresponding quantitation. Full size image Second, we used the model to simulate the steady-state abundances of IκB-bound NFκB dimers in wild-type cells; this resulted in the prediction that the majority of A:A homodimers are associated with IκBβ for the probable, but not the improbable affinity sets ( Fig. 5d ). Further, the majority of A:50 dimers were predicted to be associated with IκBα, but in some, the primary interaction partner was IκBβ ( Fig. 5d ). To test this prediction we prepared cytoplasmic extracts from unstimulated MEFs that contain latent IκB–NFκB complexes. The ionic detergent deoxycholate is known to disrupt IκB–NFκB interactions while leaving the dimer intact and capable of binding DNA [19] , thereby revealing both latent RelA homo- and heterodimers ( Fig. 5e , lane 2). By prior immunodepleting IκBα or IκBβ, we found that IκBβ (>50%) is indeed the primary interaction partner for the A:A homodimer (lane 6), whereas IκBα depletion left the A:A homodimer largely intact (lane 4). In addition, we found that IκBα is the primary interaction partner (>50%) for the A:50 heterodimer (lane 4), although some A:50 is bound to IκBβ as well (lane 6). On the basis of these data, we were able to narrow the probable parameter range by excluding parameter sets that did not satisfy the experimentally determined IκB–NFκB interactions ( Supplementary Table 5 ). Finally, we asked whether IκBβ is in fact required for A:A homodimer generation. Computational simulations with the probable affinity sets predicted a dramatic decrease (<20% of wild type) in A:A homodimer abundance in IκBβ-deficient but not in IκBα-deficient cells ( Fig. 5f ). Improbable parameter affinity sets yielded variable amounts of A:A homodimer abundance in the three genotypes. Our experimental analysis supported the probable affinity sets’ predictions: IκBβ-deficient cells showed a dramatic drop (<2% of wild type) in the A:A homodimer abundance as revealed by deoxycholate treatment of cytoplasmic extracts, whereas IκBα deficiency did not appear to alter the A:A homodimer repertoire (>97% of wild type; Fig. 5g ). We then determined which of the parameter sets passed the above three tests. Remarkably, none of the improbable parameters allowed for correct predictions, while two parameter sets from the initially determined probable range did ( Supplementary Table 5 ). These three model-directed experimental studies thus support the notion that a high affinity for the A:A homodimer endows IκBβ with a stabilizing role in the abundance of the A:A homodimer. Interestingly, two NFκB target genes ( MIP-2 and TNF α), whose expression was found to be mediated by RelA:RelA homodimers, showed a marked reduction in IκBβ-deficient cells (particularly at late time points), whereas expression of RelA:p50 target genes was not reduced but elevated instead ( Supplementary Fig. 3 ). IκBβ counters monomer competition and rescues RelA homodimer Our work thus far has identified two system properties that control the RelA:RelA abundance: monomer competition and IκBβ-mediated stabilization. These mechanisms have opposing effects on RelA:RelA homodimer abundance, and so we examined their relationship to each other by simulating the effect of IκBβ deficiency in the context of p50-containing or p50-deficient cells. In p50-deficient cells, compensation by p52 is observed but remains incomplete [7] ; in our simulations we account for that with a 30-fold reduction in p50 synthesis rates (qualitatively similar results were obtained with a range of synthesis rates; Fig. 6a ). We find that loss of IκBβ in p50-deficient cells result in lower A:A abundance, although the A:A homodimer remains detectable in contrast to results in p50-containing cells, in which A:A abundance was more IκBβ-dependent ( Fig. 5f,g ). 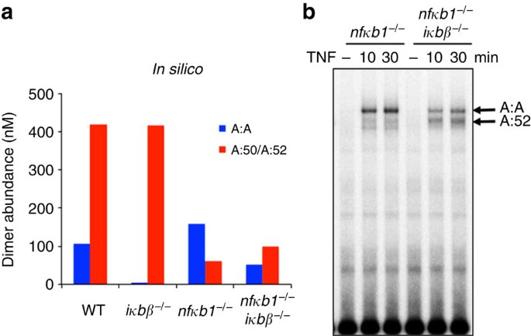Figure 6: IκBβ is important in RelA homodimer formation. (a) Bar graph depicting the simulation results of NFκB dimer abundances in wild-type, IκBβ-deficient, p50-deficient and IκBβ/p50 doubly deficient MEFs. Compensation by p52 in p50-deficient cells was simulated by allowing for synthesis of a p50-like molecular species. (b) EMSA of nuclear extracts prepared from p50-deficient and p50/IκBβ-deficient MEFs treated with TNF at 10 and 30 min. In the absence of p50-mediated monomer competition, the RelA:RelA homodimer is highly abundant, even in the absence of IκBβ. Data shown are representative of three independent experiments. Figure 6: IκBβ is important in RelA homodimer formation. ( a ) Bar graph depicting the simulation results of NFκB dimer abundances in wild-type, IκBβ-deficient, p50-deficient and IκBβ/p50 doubly deficient MEFs. Compensation by p52 in p50-deficient cells was simulated by allowing for synthesis of a p50-like molecular species. ( b ) EMSA of nuclear extracts prepared from p50-deficient and p50/IκBβ-deficient MEFs treated with TNF at 10 and 30 min. In the absence of p50-mediated monomer competition, the RelA:RelA homodimer is highly abundant, even in the absence of IκBβ. Data shown are representative of three independent experiments. Full size image To test the validity of this model prediction, we generated p50/IκBβ-doubly-deficient MEFs and compared relative abundances of RelA homodimers as determined using electrophoretic mobility shift assays (EMSA; Figs 1c and 6b ). We found that in good agreement with the model predictions, IκBβ deficiency results in a lower A:A abundance, but that detectable levels of A:A homodimer remained. Thus, both our modelling and experimental results support the notion that IκBβ controls A:A abundance, and further suggest that IκBβ plays a key role in neutralizing the effect of monomer competition on the abundance of the low-affinity A:A homodimer. IκBα controls the dynamics of both RelA-containing dimers The described mathematical model recapitulates the functions of the Rel-NFκB dimer generation module in generating the latent NFκB dimer repertoire in unstimulated fibroblasts. To study stimulus-induced dynamic regulation of the generation, activation and inactivation of RelA homo- and heterodimers, we connected this model with a well-tested model of the IκB–NFκB signalling module [20] to generate Model 4 ( Fig. 7a , Supplementary Fig. 4a , Supplementary Table 4 , Supplementary Table 5 , Supplementary Table 6 , Supplementary Note 4 ). 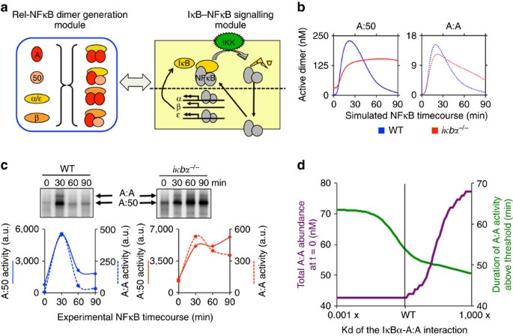Figure 7: While IκBβ regulates NFκB-RelA homodimer generation, IκBα regulates its signalling. (a) A schematic showing the linking of the Rel-NFκB dimer generation module and the IκB–NFκB signalling module20to simulate stimulus-induced activation of multiple NFκB dimers. IκBα, IκBβ and IκBɛ interact with A:A and A:50 dimers as described inFig. 5a. A detailed model schematic is shown inSupplementary Fig. 5a. (b) Computational time course simulations of TNF-stimulated nuclear DNA-binding activity of the indicated NFκB dimers A:50 (left, solid lines) and A:A (right, dashed lines) in wild-type (blue) and IκBα-deficient (red) MEFs. Both dimer activities exhibit post-induction repression mediated by IκBα. (c) EMSAs (top panels) of nuclear extracts of wild-type and IκBα-deficient MEFs prepared from TNF-stimulated cells at 30, 60 and 90 min. Quantitation (bottom panels) of the A:50 (solid lines) A:A and A:50 (dashed lines) NFκB dimers show prolonged activation in IκBα-deficient (right, red) as compared with wild-type (left, blue) MEFs. Shown is a representative of at least three independent experiments. (d) Computational simulations of A:A abundance (green) and duration of TNF-induced A:A activity (purple) as a function of the interaction affinity between IκBα and the A:A. These simulations were performed with the integrated model described ina, and they show that a lowerKdwould allow IκBα to contribute to A:A generation, while a higherKdwould reduce IκBα’s ability to terminate TNF-induced A:A activity. Figure 7: While IκBβ regulates NFκB-RelA homodimer generation, IκBα regulates its signalling. ( a ) A schematic showing the linking of the Rel-NFκB dimer generation module and the IκB–NFκB signalling module [20] to simulate stimulus-induced activation of multiple NFκB dimers. IκBα, IκBβ and IκBɛ interact with A:A and A:50 dimers as described in Fig. 5a . A detailed model schematic is shown in Supplementary Fig. 5a . ( b ) Computational time course simulations of TNF-stimulated nuclear DNA-binding activity of the indicated NFκB dimers A:50 (left, solid lines) and A:A (right, dashed lines) in wild-type (blue) and IκBα-deficient (red) MEFs. Both dimer activities exhibit post-induction repression mediated by IκBα. ( c ) EMSAs (top panels) of nuclear extracts of wild-type and IκBα-deficient MEFs prepared from TNF-stimulated cells at 30, 60 and 90 min. Quantitation (bottom panels) of the A:50 (solid lines) A:A and A:50 (dashed lines) NFκB dimers show prolonged activation in IκBα-deficient (right, red) as compared with wild-type (left, blue) MEFs. Shown is a representative of at least three independent experiments. ( d ) Computational simulations of A:A abundance (green) and duration of TNF-induced A:A activity (purple) as a function of the interaction affinity between IκBα and the A:A. These simulations were performed with the integrated model described in a , and they show that a lower K d would allow IκBα to contribute to A:A generation, while a higher K d would reduce IκBα’s ability to terminate TNF-induced A:A activity. Full size image A hallmark of NFκB signalling is negative feedback control mediated by IκBα that ensures post-induction repression of RelA:p50 activity following transient exposure to inflammatory cytokines [20] , [21] . To test whether the resulting model recapitulates the signalling dynamics of two NFκB dimers, we simulated TNF-induced signalling. Model simulations showed transient activation of both dimers in wild-type cells with relative abundances that are supported by experimental measurements of both dimers. Post-induction repression was mediated by IκBα, as i κ b α −/− MEFs showed sustained activity in both computational ( Fig. 7b ) and experimental studies ( Fig. 7c ), not only of the A:50 heterodimer, but also of the A:A homodimer. The sustained A:A homodimer activity in i κ b α −/− MEFs is not due to an increase in IκBβ protein levels ( Supplementary Fig. 4b ), but rather arises from the loss of negative feedback regulation of IκBα. While previous work has demonstrated the critical role of IκBα in the dynamic control of RelA:p50, our simulation and experimental results provide evidence that IκBα plays a role in the dynamic control of RelA:RelA activity as well. We were curious how it could be possible that IκBα is the key dynamic regulator of A:A activity but does not contribute substantially to A:A homodimer generation. We investigated these two roles as a function of the affinity between IκBα and the A:A homodimer. We simulated both the basal abundance of the A:A homodimer and the duration of A:A homodimer activity above the threshold of a 50% of maximum activity ( Supplementary Fig. 4c ) as a function IκBα-A:A homodimer affinities over a thousandfold range ( Fig. 7d ). We found that lowering the IκBα-A:A affinity would prolong A:A homodimer activity following transient stimulation, but have little impact on A:A abundance; however, increasing the affinity would increase the basal abundance of the A:A homodimer. We thus conclude that the IκBα affinity for the A:A homodimer is tuned to be low enough that IκBα does not function within the Rel-NFκB dimer generation module, but high enough so that it functions within the IκB–NFκB signalling module to control the dynamics of A:A activity. The described work reveals a novel and specific function for IκBβ. IκBs are named ‘inhibitors of NFκB’ because they are capable of inhibiting NFκB DNA-binding activity in cell-free in vitro assays [19] , and IκBβ was identified in that same manner [22] . However, we show here that in vivo IκBβ functions primarily as a positive regulator of NFκB dimer generation. Whereas the RelA:p50 dimers can readily form, owing to a high dimerization affinity, RelA:RelA homodimer formation requires the stabilizing influence of IκBβ. These distinct functions of IκBβ and other IκBs explain the phenotypes observed in knockout mice. Previous studies of the IκB–NFκB signalling module revealed that negative feedback by IκBα, IκBɛ and IκBδ shape the dynamics of NFκB activity in response to stimuli [12] , [20] , [21] , [23] , [24] , [25] . Indeed, prolonged NFκB activity leads to a severe hyperinflammatory phenotype in IκBα-deficient mice, and to hyperproliferation in B cells lacking IκBɛ (ref. 26 ) or IκBδ (ref. 36 ). However, IκBβ-deficient mice were recently reported to have hypoinflammatory responses, reduced expression of TNF and resistant to endotoxic shock and collagen-induced arthritis [5] , [27] . We show here that IκBβ-deficient fibroblasts lack one member of the NFκB dimer family, namely the homodimer of the potent activator RelA ( Fig. 3 ). Similar resultant RelA:RelA and RelA:cRel deficiency has been observed in i κ b β −/− macrophages [5] . Previously established mathematical models of the IκB–NFκB signalling module are unable to account for this phenotype. These models assume a constant amount of NFκB dimer as a given quantity, and calculate the control of its subcellular localization and DNA-binding activity as a function of dynamically regulated IκB degradation and re-synthesis. Here we have constructed a model for the Rel-NFκB dimer generation module and parameterized based on biophysical measurements of recombinant proteins and a series of iterative cycles of prediction and in vivo measurements. Our work reveals that IκBβ is critical for NFκB RelA:RelA homodimers in MEFs, whose spontaneous generation is challenged not only by poor intrinsic dimer affinities, but also by competition with the high-affinity heterodimerization partner p50. A key feature of IκBβ function is an unusually high affinity for RelA:RelA homodimers (3.2 pM). As recombinant IκBβ is not monodispersed in cell-free systems, this model-aided interpretation of cellular measurements cannot be tested directly. While subnanomolar dissociation constants have previously been reported for other protein–protein interactions [28] , it may be prudent to reconsider the simplifying assumption of the coarse-grained model formulation, in which IκBβ interacts only with the pre-formed dimer. Instead, IκBβ might be able to bind monomers sequentially ( Supplementary Fig. 5a ), in which case IκBβ may be considered a bona fide chaperone for RelA:RelA homodimer formation. Whereas the single-step reaction scheme in the original model is + A ↔ A 2 + B ↔ A 2 B , defining dissociation constants as and , the two-step reaction scheme would be A + B ↔ AB + A ↔ A 2 B , defining dissociation constants , and . Whereas Kd 1 and Kd 2 were determined to be 800 nM and 3.2 × 10 − 3 nM, respectively, in the two-step model, Kd 3 is inversely proportional to Kd 4 ( Supplementary Fig. 5b ). Thus, a two-step model would yield interaction constants in the micro- and nanomolar ranges that are more commonly observed within bimolecular interactions. In addition to IκBβ’s described role within the Rel-NFκB dimer generation module, a hypophosphorylated IκBβ has also been shown to have nuclear functions in macrophages in protecting promoter-bound NFκB from IκBα-mediated negative feedback [29] . Resistance to negative feedback may be imparted particularly to those NFκB dimers (for example, A:A and RelA:cRel) that show high affinity for IκBβ (refs 5 , 27 ). As such, both the proposed nuclear function and the here-described chaperone function are a consequence of the high affinity for specific dimers revealed through our iterative experimental and computational study. The parameterization of computational models is a recognized challenge of systems biology. Whereas strategies have been developed to parameterize mathematical synthesis and degradation expressions, as well as those describing enzymatic functions within cells, the interactions between proteins are rarely quantitatively addressed. Ex vivo , affinity and kinetic rate constants can be determined for the interaction of recombinant proteins; however, the in vivo relevance of such constants is limited by the difficulties of producing recombinant full-length proteins with appropriate post-translational modifications. Here we exploited the fact the IκB abundance is a function of its interaction with NFκB (ref. 12 ; Fig. 2b ) and employed computational modelling in order to derive in vivo interaction affinities from immunoblot quantifications. Interestingly, it was previously observed that RelA deficiency results in IκBβ deficiency [30] , [31] , and such obligate interactions are not rare [32] , [33] , suggesting that our model parameterization strategy may be employed for other biological systems. We described the Rel-NFκB dimer generation module and the IκB–NFκB signalling module as distinct but there are of course numerous interactions. At a minimum, we may consider that IκBβ, within the Rel-NFκB dimer generation module, functions as a ‘licensing factor’ for subsequent dynamic control by IκBα. The distinct functions by these structurally homologous proteins are on the basis of both their specific protein-interaction constants, and on their distinct dynamic degradation and synthesis control. Indeed, the regulatory utility of such ‘hand-off’ or ‘relay control’ network motifs, based on kinetic differences between family members, may be a driver of the expansion of protein families. Computational modelling Four computational models were constructed for this study. Models 1–3 ( Supplementary Note 1–3 ) address how NFκB dimers are generated from RelA and p50 NFκB monomers and how interactions with two IκB isoforms may affect the abundance of these dimers; model 4 addresses how nuclear localization of these NFκB dimers is induced and regulated following TNF-induced IKK activation. Model 1 ( Fig. 1a , Supplementary Note 1 ) contains RelA and p50, which form three NFκB dimers: RelA:A, RelA:p50 and p50:p50. The rate constants for the parameters in these equations are found in Supplementary Table 1 . Model 2 ( Fig. 3a , Supplementary Note 2 ) is based on model 1 above. A generic IκB can complex with RelA:A and RelA:p50. The p50:p50 dimer has not been demonstrated to bind to IκB, so that interaction is excluded from this model. We assume no degradation of the IκB–NFκB complex or the NFκB dimer from the complex; the dimer may dissociate or IκB may degraded and release the NFκB dimer. The rate constants for the parameters in these equations are found in Supplementary Table 2 . Model 3 ( Fig. 5a , Supplementary Note 3 ) is based on Model 2. IκBα/ɛ and IκBβ are the specific IκBs in the model, which can complex with RelA:A and RelA:p50. For simplicity, IκBα and IκBɛ are assumed to have the same molecular interaction characteristics and are treated as a single IκB species. The rate constants for the parameters in these equations are found in Supplementary Table 3 . Parameterization of the model required exploration of the parameter space for IκB–NFκB affinities and determining the likelihood of each set of parameter values (see results Fig. 4b ). Further parameterization involved additional experimental data ( Fig. 5 ) in order to eliminate nonconforming parameter sets (see Supplementary Table 5 ). Model 4 ( Fig. 7a , Supplementary Table 4 ) appends previously published IκB–NFκB signalling models [25] , [34] with the reactions that govern NFκB dimer generation and dimer–IκB interactions as described in model 3; however, IκBα and IκBβ are explicitly enumerated. The complete new model contains 40 species and 110 reactions governed by 65 parameters ( Supplementary Table 4 ). IκB–NFκB affinities were determined based on a series of experimental data that had to be satisfied (see Supplementary Table 5 ); parameterization included basal protein abundance measurements ( Supplementary Table 6 ). The model ODEs were solved numerically using MATLAB version R2013a (The MathWorks Inc.) with subroutine ode15s , a variable order, multistep solver. The system was allowed to equilibrate from starting conditions to a steady state, defined as showing no concentration changes greater than 1% over a period of 4,000 min. Stimulus-induced perturbation from the steady state of Model 4 was accomplished by direct modulation of IKK activity via a numerical input curve representing TNF stimulation (adapted from ref. 20 ). Code Availability MATLAB code files are available on request. Deriving IκB–NFκB affinities Model 2 was used to calculate the IκB abundances in RelA:p50-deficient and RelA:RelA-deficient cells using NFκB dimerization affinities (determined by 31 sets of d parameters for homodimers and 31 sets of heterodimers) and IκB–NFκB interaction affinities (determined by 61 sets of di parameters for IκBα and 61 for IκBβ). NFκB dimerization affinities were measured with an assumed variance of twofold, and so each IκB abundance in each cell could be associated with a probability. These were intersected with the experimentally determined distributions of IκB abundances (defined by mean and s.d. ), allowing us to determine the probability (based on available experimental data) that a specific set of the 3,575,881 possible parameter sets is correct. The probabilities for IκB–NFκB interaction affinities are shown in Fig. 4b . Specific sets of probable and improbable parameter combinations were further tested in Fig. 5 against various experimentally determined outcomes to narrow down the most probably parameter sets. Cell culture Immortalized MEFs were prepared and cultured as previously described [21] , [23] . Briefly, cells were grown to confluence in Dulbecco’s Modified Eagle’s Medium supplemented with 10% bovine calf serum, 1% penicillin–streptomycin and 1% L-Glutamine. Stimulations were performed using 1 ng ml −1 TNF (Roche). The cell lines used were as follows: wild-type (ref. 21 ), iκbβ −/− (ref. 23 ), iκbα −/− iκbɛ −/− (ref. 21 ), iκbα −/− iκbβ −/− iκbɛ −/− (ref. 12 ), rela −/− (ref. 7 ), rela −/− crel −/− nfkb1 −/− (ref. 12 ), nfkb1 −/− nfkb2 −/− (ref. 7 ). crel −/− relb −/− nfkb1 −/− nfkb2 −/− knockouts were generated from E12.5−14.5 embryos and immortalized following the 3T3 protocol. Biochemistry EMSA [21] , deoxycholate (DOC)+EMSA [24] , EMSA supershift [35] , wild-type+mutant oligo competition EMSA [7] , immunodepletion, RNase Protection Assay [23] and immunoblotting [21] were performed as previously described. Briefly, for EMSA, nuclei were collected by hypotonic lysis and resuspended in 30 μl NE buffer (250 mM Tris pH 7.8, 60 mM KCl, 1 mM EDTA, with freshly added 1 mM dithiothreitol, 1 mM phenylmethylsulfonyl fluoride (PMSF)) and lysed by three freeze-thaw cycles. Nuclear lysates were cleared by 14,000 g centrifugation and adjusted to 1 μg μl −1 total protein concentration. Total nuclear protein (2 μg) was incubated at room temperature for 15 min with 0.1 pmoles of P32-labelled 34 bp double-stranded oligonucleotide containing a consensus κB site (5′- AGCTTGCTACAA GGGACTTTCC GCTGTCTACTTT -3′) in 3 μl binding buffer (10 mM Tris-Cl pH 7.5, 50 mM NaCl, 10% glycerol, 1% NP-40, 1 mM EDTA, 0.1 μg μl −1 polydIdC). Complexes were resolved on a nondenaturing gel and visualized using a Typhoon Scanner (GE Healthcare Life Sciences). For DOC sensitivity, 2 μg of nuclear extract was treated with DOC to a final concentration of 0.8% for 30 min and subsequently subjected to EMSA analysis. For supershifts, nuclear extracts were incubated with indicated antibody cocktails for 20 min on ice before probe incubation followed by resolution on nondenaturing gel. For wt-mutant competition EMSA, nuclear extracts were incubated with 100-fold molar excess of wt and mutant κB probes and resolved as before. For RNase Protection assay, total RNA was made from confluent serum-starved fibroblasts using Trizol-Reagent (Ambion by Life Technologies). RNase Protection assay was performed with 5 μg RNA using Riboquant probe set mCK-5 (Pharmingen) according to the manufacturer’s instructions. For whole-cell western blots, cells were lysed within six-well plates using SDS–PAGE sample buffer, resolved on acrylamide gels, transferred to polyvinylidene difluoride membranes and probed with specified antibodies. IκBα (sc-371, 1:5,000), IκBβ (sc-946, 1:5,000 for immunoblot and sc-969, 1:20, for immunodepletion), RelA (sc-372, 1:5,000) antibodies were provided by Santa Cruz Biotechnology. p50 N-terminal antisera (1:10,000) was a generous gift from Nancy Rice. How to cite this article: Tsui, R. et al . IκBβ enhances the generation of the low-affinity NFκB/RelA homodimer. Nat. Commun. 6:7068 doi: 10.1038/ncomms8068 (2015).